Identification and optimization of small-molecule agonists of the human relaxin hormone receptor RXFP1 The anti-fibrotic, vasodilatory and pro-angiogenic therapeutic properties of recombinant relaxin peptide hormone have been investigated in several diseases, and recent clinical trial data has shown benefit in treating acute heart failure. However, the remodelling capacity of these peptide hormones is difficult to study in chronic settings because of their short half-life and the need for intravenous administration. Here we present the first small-molecule series of human relaxin/insulin-like family peptide receptor 1 agonists. These molecules display similar efficacy as the natural hormone in several functional assays. Mutagenesis studies indicate that the small molecules activate relaxin receptor through an allosteric site. These compounds have excellent physical and in vivo pharmacokinetic properties to support further investigation of relaxin biology and animal efficacy studies of the therapeutic benefits of relaxin/insulin-like family peptide receptor 1 activation. Despite great advances in medical science, 1 of every 2.9 deaths in the United States is due to cardiovascular disease [1] . Each year about 795,000 people experience a new or recurrent stroke, and one in nine death certificates in the United States mention heart failure. In addition, 33.5% of US adults over 20 years of age have hypertension [1] . These statistics clearly illustrate both the grave need for more effective treatments and the limitations of current therapies to address cardiovascular disease in general and acute heart failure in particular. The peptide hormone relaxin was discovered in 1926 as a hormone of pregnancy [2] , due to its relaxation effects on pubic ligaments (hence the name) and softening the cervix to facilitate parturition [3] . It has been shown that concentration of relaxin in blood rises during the first trimester of pregnancy, promoting cardiovascular and renal adjustments to meet the increased nutritional demands of the growing fetus, and the elevated requirements for renal clearance of metabolic wastes [4] . Relaxin induces a 20% increase in cardiac output, 30% decrease in systemic vascular resistance, 30% increase in global arterial compliance and 45% increase in renal blood flow during pregnancy [5] . Numerous clinical and nonclinical studies using this hormone have now recapitulated these cardiovascular effects in both males and females, demonstrating its potential pharmacological utility in modulating cardiovascular and renal function. The clinically observed physiological effects of relaxin are mediated though its interaction with the G-protein-coupled receptor, relaxin/insulin-like family peptide receptor 1 (RXFP1), leading to the modulation of several signal transduction pathways [6] . Activation of RXFP1 by relaxin induces: (1) upregulation of the endothelin system that leads to vasodilation; (2) extracellular matrix remodelling through regulation of collagen deposition, matrix metalloproteinase and tissue inhibitor of metalloproteinase expression, and overall tissue homoeostasis; (3) a moderation of inflammation by reducing levels of inflammatory cytokines, such as tumour necrosis factor-alpha and transforming growth factor beta; and (4) angiogenesis by activating transcription of vascular endothelial growth factor ( VEGF ) [6] , [7] , [8] . The understanding of the biological effects of RXFP1 activation by relaxin has led to the evaluation of relaxin as a pharmacological agent for the treatment of patients with acute heart failure [9] , [10] , preeclampsia [11] and hypertensive diseases [12] , [13] . Given its anti-inflammatory and extracellular matrix remodelling function, several clinical trials have also evaluated the potential of relaxin as treatment for scleroderma, cervical ripening, fibromyalgia and orthodontics [8] . A similar anti-inflammatory and remodelling need also exists for cardiac rehabilitation. None of the current methodologies, such as surgery, medical devices or approved medications (angiotensin-converting enzyme inhibitors, angiotensin II receptor blockers, digoxin, beta blockers and aldosterone antagonists), are able to prevent the development of heart tissue scar after acute heart failure, or repair heart tissue after damage is incurred. The anti-fibrotic and remodelling properties of relaxin [9] , [14] , together with its capacity to normalize blood pressure, increase blood and renal flow [15] , seem to be ideal for the treatment of patients with cardiovascular diseases. Clinical trial data support this theory [9] , [16] . Relaxin relieves systemic and renal vasoconstriction and increases vascular compliance, including normalization of high blood pressure, reduction of pulmonary capillary wedge pressure, increase of cardiac output, increase renal blood flow, natriuresis and decongestion [17] . Recent data from the RELAX-AHF phase III clinical trial showed that the early administration of serelaxin, a recombinant analogue of the natural hormone, reduced overall mortality at 6 months and promoted a more rapid relief of congestion with fewer signs of organ damage during the initial days after admission [9] , [10] . In addition, animal pharmacology data indicate that relaxin hormone has anti-inflammatory and cardiac protection effects, including reduction of myocardial ischaemia and reperfusion injury, increase of wound healing, reduction of ventricular fibrosis [14] and increase of endothelial progenitor cell mobilization [18] . Recombinant relaxin hormone has produced promising responses in clinical trials for the treatment of heart failure and is close to commercialization [9] . However, the peptide is difficult to administer as a chronic therapy. The half-life of this peptide hormone is <10 min and it has to be administrated intravenously [13] . The development of small-molecule agonists of RXFP1 as an alternative to recombinant hormone would have numerous benefits and will enable the investigation of additional therapeutic applications that may require chronic administration. In this article, we report the first series of small-molecule agonists of RXFP1. These small molecules are potent, highly selective, orally bioavailable and easy to synthesize. Identification of hits as small-molecule agonists of RXFP1 More than 350,000 compounds of the Molecular Libraries Probe Center Network library [19] were tested in a quantitative high-throughput screening [20] campaign searching for small-molecule agonists of RXFP1, by measuring the ability of compounds to elevate cyclic adenosine monophosphate (cAMP) levels in a HEK293 cell line stably transfected with human RXFP1 [21] . Maximal cAMP signal was established by treatment with porcine relaxin (1.66 nM) or the adenylyl cyclase activator forskolin (57 μM). Confirmed active compounds were further interrogated using the naive parental HEK293 cell line and cells transfected with the related receptors insulin-like 3 peptide receptor, RXFP2 , or arginine vasopressin receptor 1B, AVPR1B , using the same cAMP detection kit as screens for selectivity and to eliminate compounds which non-specifically increase the cAMP signal through an RXFP1-independent mechanism. Two molecules 1 and 2 with modest activity in the primary screen were validated using these counter-screen assays [21] and then resynthesized in-house. Both confirmed hits displayed similarities in their chemical scaffold containing a 2-acetamido- N -phenylbenzamide core in their structures ( Fig. 1 , in blue). 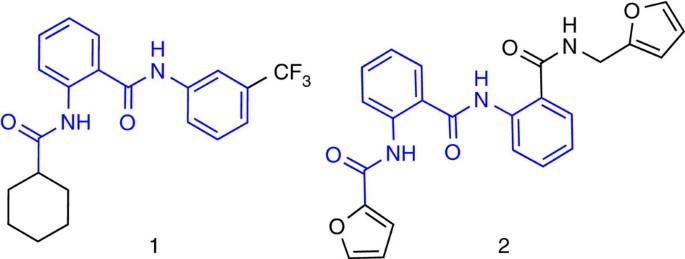Figure 1: Chemical structures of hit molecules 1 and 2 identified in a RXFP1 cAMP primary screening assay. Both molecules share a common chemical scaffold containing a core substructure of 2-acetamido-N-phenylbenzamide (in blue). Figure 1: Chemical structures of hit molecules 1 and 2 identified in a RXFP1 cAMP primary screening assay. Both molecules share a common chemical scaffold containing a core substructure of 2-acetamido- N -phenylbenzamide (in blue). Full size image Hit-to-lead medicinal chemistry optimization The initial screening was followed up by an extensive structure activity relationship campaign to improve the potency, efficacy and physical properties of the compounds ( Fig. 2 ; Supplementary Table S1 ). Compound activity is reported through two measurements: EC 50 (concentration necessary to reach 50% of the maximum cAMP signal produced by the molecule) and maximum response (efficacy, corresponding with the level of cAMP elevation normalized to relaxin control). Both EC 50 and maximum response were evaluated and optimized through these efforts. Our studies on the aniline ring indicated the importance of a hydrophobic functional group having the proper field effect [22] at the meta -position of this aromatic ring, with a trifluoromethylsulfonyl group providing the best activity. Meta -substituents with incremental field-effect values at this position (SO 2 CF 3 , F=0.73; SCF 3 , F=0.35; and CF 3 , F=0.38) [22] provide increasingly potent activity. We also investigated the impact of modifying the cyclohexane ring moiety and found that aromatic replacements, especially those with an alkoxy aliphatic chain in ortho -position, increased compound potency. Finally, most substituents and replacement modifications of the middle phenyl ring core and amide functional groups produced analogues with the same or lower activity than the corresponding parent compound. 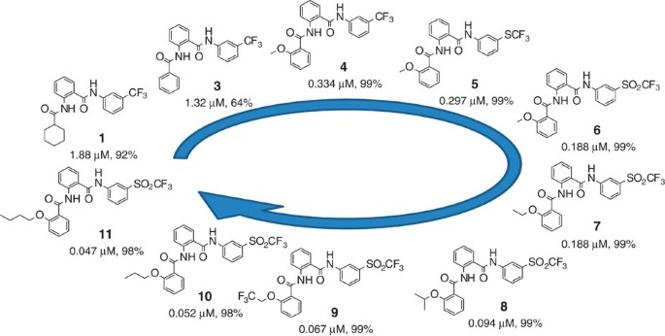Figure 2: Structure activity relationship optimization campaign. Ten representative compounds,1and3–11, highlight the key steps in the hit-to-lead evolution. The EC50and relative activity for each compound are shown using the RXFP1 primary screening assay. 100% relative activity was normalized to 57.7 μM forskolin stimulation, and 0% relative activity was normalized to compound vehicle control (0.58% DMSO). Complete concentration-response data are also provided (Supplementary Fig. S1). Figure 2: Structure activity relationship optimization campaign. Ten representative compounds, 1 and 3 – 11 , highlight the key steps in the hit-to-lead evolution. The EC 50 and relative activity for each compound are shown using the RXFP1 primary screening assay. 100% relative activity was normalized to 57.7 μM forskolin stimulation, and 0% relative activity was normalized to compound vehicle control (0.58% DMSO). Complete concentration-response data are also provided ( Supplementary Fig. S1 ). Full size image Profiling of representative lead compounds Table 1 displays the profile of compounds 5 – 11 with an EC 50 <300 nM in the RXFP1 -transfected cAMP assay, and also includes their activities in a human monocytic leukaemia cell line (THP1), which endogenously expresses the RXFP1 receptor, their selectivity against HEK293 cells transfected with the receptors RXFP2 and AVPR1B , adenosine triphosphate (ATP) cytotoxicity, aqueous PBS solubility and mouse liver microsomal stability ( Supplementary Table S2 ). As expected, because of the lipophilic character of our molecules, these compounds have poor water solubility, although our most potent compounds ( 8 – 11 , EC 50 <100 nM) display a solubility of 3.3–17.0 μM, which is 49–327 times higher than their corresponding EC 50 for RXFP1 in HEK293 cells. Table 1 Profiles of potent analogues 5–11 with EC 50 <300 nM in the RXFP1-transfected HEK293 cAMP assay. Full size table Lead compounds increase VEGF expression in THP1 cells Beyond inducing elevated intracellular cAMP levels, we also evaluated the ability of the most potent compounds 5 – 11 to activate the transcription of the known relaxin target gene, VEGF , in THP1 cells [23] , [24] . The addition of 10 ng ml −1 (1.66 nM) of relaxin hormone induces a significant increase (2.4 fold) in the relative expression of VEGF mRNA as measured by quantitative real-time PCR. Similar effects were obtained in cells stimulated with compound ( Fig. 3 ). 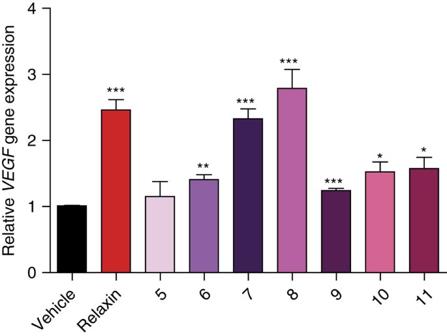Figure 3: Activation ofVEGFgene expression in THP1 cells. THP1 cells were treated with compound vehicle control (0.58% DMSO), relaxin (10 ng ml−1; 1.66 nM) or seven representative compounds5–11at 250 nM for 2 h. The level ofVEGFgene expression was measured by quantitative real-time PCR and normalized toGAPDHexpression and vehicle control as 1 (n=4 for each). All analogues other than compound5show significant (*P<0.05; **P<0.01; and ***P<0.001) upregulation ofVEGFgene expression between treatment groups and vehicle control. Scale bars, mean values±s.e.m.; statistical analysis was performed using two-tailed, Student’st-test. Figure 3: Activation of VEGF gene expression in THP1 cells. THP1 cells were treated with compound vehicle control (0.58% DMSO), relaxin (10 ng ml −1 ; 1.66 nM) or seven representative compounds 5 – 11 at 250 nM for 2 h. The level of VEGF gene expression was measured by quantitative real-time PCR and normalized to GAPDH expression and vehicle control as 1 ( n =4 for each). All analogues other than compound 5 show significant (* P <0.05; ** P <0.01; and *** P <0.001) upregulation of VEGF gene expression between treatment groups and vehicle control. Scale bars, mean values±s.e.m. ; statistical analysis was performed using two-tailed, Student’s t -test. Full size image Lead compound 8 increases cell impedance in HEK293 cells Cellular impedance was measured using xCELLigence Analyzer (Roche Diagnostics, Indianapolis, IN), which allows for continuous time-resolved measurement of cellular index without additional labelling [25] . Cells were treated with compound for 30 min. Given this short incubation time, changes in cell number were unlikely to contribute to the overall effect. The results indicate that compound 8 treatment generated a dose-dependent response similar to that of relaxin hormone ( Fig. 4a ). Neither treatment affected cell impedance in the corresponding parental HEK293 cells ( Fig. 4c ), indicating that changes in cell impedance were mediated through RXFP1. 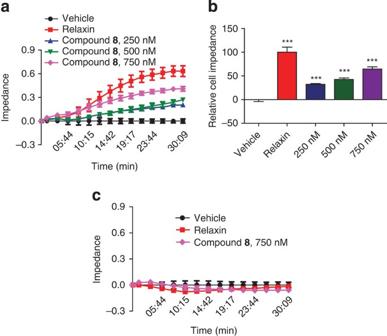Figure 4: Compound 8 exhibits concentration-dependent increase of cellular impedance inRXFP1-transfected HEK293 cells. (a) Effect of relaxin (10 ng ml−1; 1.66 nM), compared with compound8at 250 nM, 500 nM and 750 nM on cell impedance in HEK293 cells stably transfected withRXFP1(n=4 for each). The values at each point were normalized to the values of vehicle treatment. The subset of data points was used for the graph drawing. All points represent the mean values±s.e.m. (b) Relative cell impedance normalized to the relaxin treatment group (100) at 30 min after addition of relaxin or compound8. Columns represent the mean values±s.e.m. Differences, evaluated by two-tailed, Student’st-test, between treatment groups and vehicle control are significant (***P<0.001). (c) Relaxin (10 ng ml−1; 1.66 nM) and compound8at 750 nM did not affect cell impedance in parental HEK293 cells. Figure 4: Compound 8 exhibits concentration-dependent increase of cellular impedance in RXFP1 -transfected HEK293 cells. ( a ) Effect of relaxin (10 ng ml −1 ; 1.66 nM), compared with compound 8 at 250 nM, 500 nM and 750 nM on cell impedance in HEK293 cells stably transfected with RXFP1 ( n =4 for each). The values at each point were normalized to the values of vehicle treatment. The subset of data points was used for the graph drawing. All points represent the mean values±s.e.m. ( b ) Relative cell impedance normalized to the relaxin treatment group (100) at 30 min after addition of relaxin or compound 8 . Columns represent the mean values±s.e.m. Differences, evaluated by two-tailed, Student’s t -test, between treatment groups and vehicle control are significant (*** P <0.001). ( c ) Relaxin (10 ng ml −1 ; 1.66 nM) and compound 8 at 750 nM did not affect cell impedance in parental HEK293 cells. Full size image Three-dimensional conformation and stability of the lead compound 8 The minimum energy conformation of compound 8 was determined in solid state by X-ray crystallography ( Fig. 5 ; Supplementary Table S3 ) and in solution by variable temperature NMR and Nuclear Overhauser Effect (NOE) spectroscopy studies ( Supplementary Fig. S2 ). The two intramolecular hydrogen-binding interactions found in compound 8 rigidify its three-dimensional conformation, possibly contributing to its remarkable stability. Moreover, stability studies using mouse and human plasma demonstrated that compound 8 has excellent plasma stability in vitro ( Supplementary Table S4 ), with no significant decrease after 2 h of exposure. 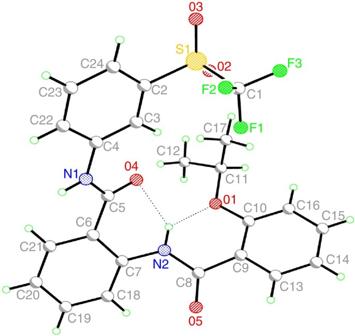Figure 5: Three-dimensional conformation of compound 8 determined by X-ray diffraction crystallography. Two intramolecular hydrogen-binding interactions (dash lines) are identified with a bond length of 2.03 and 2.12 Å, respectively. Full parameters are also provided (Supplementary Table S3). Figure 5: Three-dimensional conformation of compound 8 determined by X-ray diffraction crystallography. Two intramolecular hydrogen-binding interactions (dash lines) are identified with a bond length of 2.03 and 2.12 Å, respectively. Full parameters are also provided ( Supplementary Table S3 ). Full size image In vivo pharmacokinetic of the lead compound 8 in mice We measured the plasma and heart concentration of compound 8 in C57BL/6 mice after a single intraperitoneal administration at a dose of 30 mg kg −1 ( Fig. 6 ; Supplementary Table S5 ). Compound 8 has a long half-life in both plasma ( T 1/2 =8.56 h) and heart ( T 1/2 =7.48 h). In addition, exposure in heart was generally three to four times higher than plasma levels. Furthermore, no abnormal clinical behaviours or acute toxicity were observed in animals throughout the study. 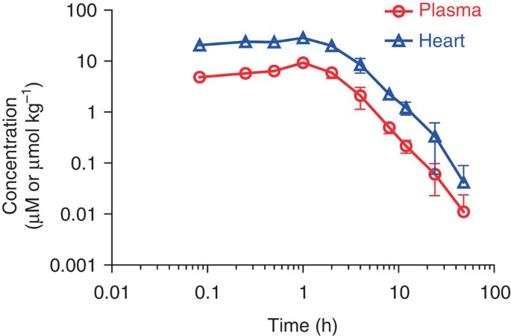Figure 6:In vivoPK profile of compound 8. Mean plasma and heart concentration-time profiles of compound8±s.e.m. after a single intraperitoneal (IP) dose of 30 mg kg−1in male C57BL/6 mice (n=3). No abnormal clinical observation was found during the in-life phase. The IP dosing formulation solution was prepared in 10% NMP+10% Solutol HS15+10% PEG400+70% saline. Full PK data and parameters are also provided (Supplementary Table S5). Figure 6: In vivo PK profile of compound 8. Mean plasma and heart concentration-time profiles of compound 8 ±s.e.m. after a single intraperitoneal (IP) dose of 30 mg kg −1 in male C57BL/6 mice ( n =3). No abnormal clinical observation was found during the in-life phase. The IP dosing formulation solution was prepared in 10% NMP+10% Solutol HS15+10% PEG400+70% saline. Full PK data and parameters are also provided ( Supplementary Table S5 ). Full size image RXFP1 region responsible for activation by compound 8 The majority of preclinical studies with relaxin peptide have been performed on mouse and rat models. Therefore, we analysed the performance of our series of agonists on HEK293 cells transfected with mouse RXFP1 (89% identity to human sequence) and found that the compounds are significantly better agonists for the human RXFP1 than for the mouse clone ( Fig. 7 ). We took advantage of this difference in species activity to map out the regions of the human receptor that determine such specificity. We tested a number of chimeric mouse/human RXFP1 constructs and found that the human receptor region of transmembrane helix 5 to extracellular loop 3 (ECL3) is required for the activation by compound 8 . Importantly, all receptor constructs responded to relaxin. Further site-specific mutagenesis studies demonstrated that the substitution of mouse ECL3 sequence with the human ECL3 resulted in full activation of the mouse receptor after treatment with compound 8 . Conversely, applying mouse 659 GT 660 / 659 DS 660 mutations to ECL3 of human receptor completely abolished compound 8 -induced cAMP activation, whereas a mouse construct with the 659 DS 660 / 659 GT 660 equivalent mutation recovered partial activity ( Fig. 7 ). 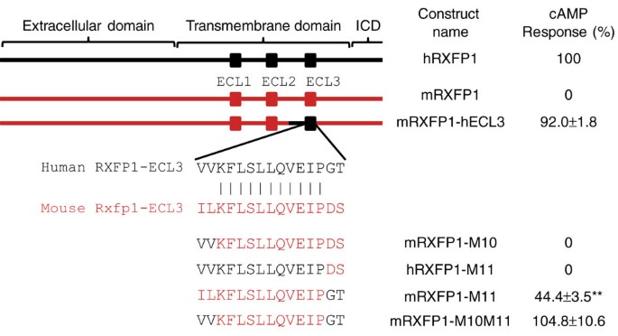Figure 7: Identification of RXFP1 region responsible for activation by compound 8. Human RXFP1 (hRXFP1 denoted for clarity in black) is fully activated (100%) after treatment with relaxin (15 nM) or compound8(66 μM). Mouse RXFP1 (mRXFP1 denoted in red) does not respond to compound8(marked as 0%) at 66 μM. RXFP1 contains extracellular, transmembrane and intracellular domains (ICDs). Using chimeric mouse–human receptors, the region responsible for RXFP1 activation by compound8was mapped to the part containing ECL3 of the transmembrane domain. Alignment of hRXFP1 and mRXFP1 shows two pairs of divergent amino acids within ECL3. The N-terminal IL to VV substitution in the mouse construct (mRXFP1-M10) did not rescue mouse receptor response, whereas C-terminal GT to DS substitution in human RXFP1 (hRXFP1-M11) abolished its compound8-dependent activation. The mouse construct with (mRXFP1-M11) mutant was partially active and the mouse receptor with humanized ECL3 (mRXFP1-M10M11) was fully active after stimulation with compound8. The cAMP response to compound8(66 μM) in cells transfected with a specific construct was normalized to the response of the same cells to relaxin (15 nM). The results represent the average of three independent experiments±s.e.m. repeated in quadruplicates. **P<0.01 versus mRXFP1 by Student’st-test. Figure 7: Identification of RXFP1 region responsible for activation by compound 8. Human RXFP1 (hRXFP1 denoted for clarity in black) is fully activated (100%) after treatment with relaxin (15 nM) or compound 8 (66 μM). Mouse RXFP1 (mRXFP1 denoted in red) does not respond to compound 8 (marked as 0%) at 66 μM. RXFP1 contains extracellular, transmembrane and intracellular domains (ICDs). Using chimeric mouse–human receptors, the region responsible for RXFP1 activation by compound 8 was mapped to the part containing ECL3 of the transmembrane domain. Alignment of hRXFP1 and mRXFP1 shows two pairs of divergent amino acids within ECL3. The N-terminal IL to VV substitution in the mouse construct (mRXFP1-M10) did not rescue mouse receptor response, whereas C-terminal GT to DS substitution in human RXFP1 (hRXFP1-M11) abolished its compound 8 -dependent activation. The mouse construct with (mRXFP1-M11) mutant was partially active and the mouse receptor with humanized ECL3 (mRXFP1-M10M11) was fully active after stimulation with compound 8 . The cAMP response to compound 8 (66 μM) in cells transfected with a specific construct was normalized to the response of the same cells to relaxin (15 nM). The results represent the average of three independent experiments±s.e.m. repeated in quadruplicates. ** P <0.01 versus mRXFP1 by Student’s t -test. Full size image We have identified the first novel series of small-molecule agonists of RXFP1 through a screening of >350,000 compound libraries in quantitative high-throughput screening format with >100-fold selectivity over RXFP2 receptor ( Fig. 1 ). Through extensive medicinal chemistry efforts, a pool of lead compounds with improved potency and selectivity were discovered ( Fig. 2 ). Analogue 3 was obtained by replacement of the cyclohexyl group in hit compound 1 with a phenyl ring. Analogue 4 was obtained from 3 by introduction of an ortho -methoxy group within this benzoic substituent. Meta -substituents with increased field-defect values on the aniline ring yield compounds 4 – 6 . Lastly, compounds 7 – 11 were produced from analogue 6 through the introduction of longer aliphatic chains within the ortho -alkoxy substituent of the benzoic ring. Optimized compounds show a remarkable increase in activity from the high micromolar EC 50 of the initial hits to potencies <50 nM ( 11 , EC 50 =47 nM, maximum response=98%). The activity of all our analogues was further tested in cAMP-response assays against RXFP2 and also counter-screened against AVPR1B. Cytotoxicity was also evaluated by measuring cellular ATP levels 72 h after treatment. Most of the analogues were inactive against RXFP2 and AVPR1B and had low cytotoxicity. These analogues also show a remarkable rodent and human microsomal stability, especially important in light of the poor metabolic stability of the recombinant hormone [26] , with intrinsic half-lives >100 min and at least 100-fold potency separation between RXFP1 activities and cytotoxicity in the same cells, measured by overall ATP cellular levels as an indicator of cell growth and viability ( Table 1 ). In addition, no activity with RXFP3, another member of the relaxin family of receptors, was detected for compound 8 (R. Bathgate, personal communication). The cAMP EC 50 of the molecules decreases only by a factor of two between RXFP1-transfected HEK293 cells and THP1 cells endogenously expressing this receptor. Differences in EC 50 among transfected and native cell lines have been previously reported for G-protein-coupled receptors and explained as function of receptor reserve, which is a measurement of the receptor occupancy required to mediate the response and amplification of the signal [27] . Transfected cell lines, with an elevated number of receptor transcripts, produce a higher expression of the receptor on the cell surface and might require less amount of compound to elicit an equivalent functional signal. Moreover, transfection efficiency is cell type dependent. Thus, differences in EC 50 depend on the cell type and expression of the receptor in transfected cells. Although VEGF stimulation seems to be dependent on cAMP activation [23] , some differences in compound activity were observed between assays measuring cAMP elevation and VEGF stimulation. The strongest effect on VEGF activation was obtained after treatment with compounds 7 and 8 . In addition to cAMP elevation, RXFP1 activation by relaxin hormone is known to stimulate other pathways including protein kinase A, protein kinase C and extracellular signal-regulated protein kinases 1 and 2 [28] . These other pathways might also contribute to the modulation of VEGF transcriptional activation. Differences in functional selectivity between members of our series or between relaxin hormone and our compounds might have an impact on VEGF expression. Our group has previously described significant differences in functional selectivity with compounds belonging to a specific chemical class for other G-protein-coupled receptors [29] . As a further confirmation that the compound effects were RXFP1 dependent, we recapitulated previous work showing that RXFP1 activation by compound 8 increases the cell impedance of transfected cells [25] . Balancing the potency, efficacy and in vitro metabolic stability properties of our analogues, we chose compound 8 for full mouse in vivo pharmacokinetic (PK) studies investigating its levels in plasma and heart upon drug administration. Upon a single intraperitoneal dose of compound 8 at 30 mg kg −1 in male C57BL/6 mice, the concentration of compound 8 in heart reached 28.6 μmol kg −1 ( C max ) within 1 h, and concentrations above its EC 50 of 200 nM in THP1 cells was maintained for a period of 12 h in plasma and more than 24 h in heart. Oral gavage and intravenous administration recapitulate the overall PK properties of compound 8 ( Supplementary Table S6 ), indicating good metabolic stability with an extended exposure, and preferential distribution towards the heart. The oral bioavailability was low (F≈14%), which we attribute to poor solubility and suboptimal formulation. Nevertheless, excellent exposure was observed at this dose. Additional formulation studies or introducing solubilizing moieties into the molecule might further improve oral bioavailability. According to the two-domain model of relaxin binding to RXFP1, the native hormone first interacts with leucine-rich repeats of extracellular domain, and then with the extracellular loops of the transmembrane domain, most probably with ECL2 [30] , [31] , [32] . This follows by an effect on the intracellular N terminus located at low-density lipoprotein class A domain that is necessary for the activation of the RXFP1 signalling. Receptors without this domain or with a mutated domain including both mutations at the calcium-binding asparagine or substituted with glutamic acid (D 58 E) bind relaxin normally but do not signal [33] . Surprisingly, compound 8 can still induce cAMP production with this latter D 58 E mutant, indicating that the receptor activation by the small molecule does not require a functional lipoprotein domain ( Supplementary Fig. S3 ). The evaluation of compound 8 up to a concentration of 30 μM was unable to displace the binding of [ 125 I]-human relaxin to human RXFP1 ( Supplementary Table S7 ). This data, in addition to our mutagenesis studies, suggest that our small-molecule agonists likely interact with an allosteric site at the ECL3 loop and act non-competitively with the natural hormone to activate RXFP1. In summary, we present the first synthetic small-molecule alternative to relaxin hormone. The described molecules show good potency, selectivity and functional activity in cell-based assays. Our structural studies show that our agonists appear to function through a novel allosteric mechanism. Optimized compounds display excellent in vitro ADME properties and in vivo PK properties with high levels of exposure for extended period of time. These molecules represent the first bioavailable small-molecule agonists of human RXFP1 and a promising series to further investigate relaxin biology and evaluate the therapeutic benefits of RXFP1 activation in chronic settings. General methods for chemistry Full experimental details and characterization data for all new compounds are included in the Supplementary Methods . Measurements of cAMP concentration cAMP assay was performed using HTRF cAMP HiRange kit (CisBio, Bedford, MA, USA). The THP1 and HEK293 cells (ATCC, Manassas, VA, USA) stably [7] , [34] or transiently transfected with human RXFP1 , RXFP2 or AVPR1B receptor were stimulated with relaxin, the compounds or forskolin for 30 min at 37 °C, 5% CO 2 , after which, 8 μl per well of each HTRF detection reagent (diluted according to assay kit directions in HTRF lysis buffer) was added. The plates were incubated for 30 min at room temperature, and the signal was read on a ViewLux (PerkinElmer, Waltham, MA, USA) or a FLUOstar Omega (BMG Labtech, Cary, NC, USA) plate readers. Nonlinear regressions to the Hill equation were performed using Prism software (GraphPad Software, San Diego, CA, USA). ATP cytotoxicity assay in HEK293-RXFP1 cells A cytotoxicity assay to measure the effect of compounds on cell viability was performed by measuring ATP levels (ATPLite; Promega, Madison, WI, USA). Cells were incubated with compounds for 72 h in growth media (DMEM 10% FBS, 1 × Pen/Strep, 0.5 mg ml −1 of G418) in 384-well format. After compound incubation, the levels of ATP in each well were measured with the addition of the ATPLite assay reagent. Nonlinear regressions to the Hill equation were performed using Prism software. Aqueous solubility and metabolic stability measurement Kinetic solubility analysis in PBS solution was performed via a fee-for-service type of contract at Analiza based upon quantitative nitrogen detection as described ( www.analiza.com ). One sample was supplied as a dimethylsulphoxide (DMSO)-dissolved stock (10 mM). A final DMSO concentration of 2.0% and maximum theoretical compound concentration of 200 μM was achieved by diluting a 6 μl aliquot of DMSO stock with 294 μl of 1 × PBS using Hamilton Starlet liquid handling and incubated directly in a Millipore solubility filter plate. Following 24 h incubation at ambient temperature (22.0–23.0 °C), the sample was vacuum filtered. The filtrate was injected into the nitrogen detector for quantification on Analiza’s Automated Discovery Workstation. The results are reported here in both μM and μg ml −1 . Three separate on-board performance indicating standards were assayed in triplicate with supplied compounds, and the results were within the acceptable range. Mouse liver microsomal stability analysis was performed via a fee-for-service type of contract by Pharmaron ( www.pharmaron.com ). The detailed protocols can be found in the Supplementary Table S2 . VEGF expression analysis The VEGF stimulation in THP1 cells was analysed by quantitative real-time PCR. A total of 400,000 THP1 cells (0.4 ml at 1 × 10 6 cells per ml) in test media (RPMI-1640 without phenol red, 0.5% FBS, 1 × Pen/Strep and 0.05 mM of 2-mercaptoethanol) were seeded in each well on a 24-well plate. After 24 h at 37 °C, 5% CO 2 , relaxin, compounds or vehicle were added for 2 h. The cells were collected and RNA was extracted using Trizol reagent (Invitrogen, Carlsbad, CA, USA) according to the manufacturer’s instructions. cDNA was synthesized using Verso cDNA kit (Thermo Scientific, Waltham, MA, USA) according to the manufacturer’s protocol. The VEGF and GAPDH gene expression were analysed using Roche LightCycler 480 (Roche Diagnostics) with the appropriate set of primers and probes spanning different exons. The relative fold change in VEGF mRNA level was calculated by the comparative C t (2 − ΔΔ C t ) method using GAPDH expression for normalization. The experiments were repeated three times in quadruplicates. The data were analysed by Student’s t -test. Cell impedance assay in HEK293-RXFP1 cells The cell line stably transfected with RXFP1 receptor and the parental HEK293 cells were used for the cell impedance assay. Cellular impedance was measured using a Roche DP RCTA xCELLigence Analyzer (Roche Diagnostics) on E-Plates as described before [35] . Delta cellular indices were calculated as the change of impedance at a given time t , from the time of compound addition (CI compound ): ΔCI t =CI t −CI compound . Impedance at each time point was then normalized to the average of quadruplicate CI of cells treated with vehicle (V1, V2, V3 and V4), to calculate normalized delta cell index NΔCI= (CI t −CI compound )/average [ΔCI V1 , ΔCI V2 , ΔCI V3 , ΔCI V4 ]. A total of 20,000 cells were added per well in a volume of 100 μl test media and allowed to sediment at room temperature for 30 min. The plate was placed into xCELLigence RTCA DP Instrument in the CO 2 incubator overnight to allow the cells to attach. Relaxin (10 ng ml −1 ; 1.66 nM), vehicle or compound at different concentrations (250, 500 and 750 nM) were added to the wells, and the cellular impedance was measured every 30 s for 30 min. The graphs depicted in this manuscript were prepared in Prizm software using a subset of data points acquired by the xCELLigence software. The data were analysed by two-tailed, Student’s t -test using Prism software. Study of chimeric and site-specific mutant receptors Full-length human RXFP1 in pCR3.1 was used for production of site-specific and chimeric constructs. Mouse RXFP1 cDNA clone was a kind gift from Dr R. A. D. Bathgate (Howard Florey Institute, Melbourne, Australia). Chimeric receptors containing parts of mouse or human sequence were generated using overlap PCR. Site-specific human and mouse mutant receptors were generated by conventional method using long-range PCR with overlapping primers containing mutated nucleotide sites, then digested by Dpn I and transformed into competent cells. The cDNA inserts of the resulted clones were completely sequenced to confirm the correct substitutions. Transient transfections of HEK293 cells were performed using Lipofectamine 2000 transfection reagent (Invitrogen) according to the manufacturer’s instructions. Cells transiently expressing the receptors were used within 48 h of transfection in cAMP assay as described above. Cells expressing each construct were treated with different concentrations of relaxin or compound 8 in the same experiment in quadruplicates. Each construct was tested at least three times. Accession codes: The X-ray crystallographic coordinates for structure reported in this article have been deposited at the Cambridge Crystallographic Data Centre (CCDC), under deposition number CCDC 933133. These data can be obtained free of charge from the Cambridge Crystallographic Data Centre via www.ccdc.cam.ac.uk/data_request/cif How to cite this article: Xiao, J. et al. Identification and optimization of small-molecule agonists of the human relaxin hormone receptor RXFP1. Nat. Commun. 4:1953 doi: 10.1038/ncomms2953 (2013).